Comparative transcriptome analysis reveals vertebrate phylotypic period during organogenesis One of the central issues in evolutionary developmental biology is how we can formulate the relationships between evolutionary and developmental processes. Two major models have been proposed: the 'funnel-like' model, in which the earliest embryo shows the most conserved morphological pattern, followed by diversifying later stages, and the 'hourglass' model, in which constraints are imposed to conserve organogenesis stages, which is called the phylotypic period. Here we perform a quantitative comparative transcriptome analysis of several model vertebrate embryos and show that the pharyngula stage is most conserved, whereas earlier and later stages are rather divergent. These results allow us to predict approximate developmental timetables between different species, and indicate that pharyngula embryos have the most conserved gene expression profiles, which may be the source of the basic body plan of vertebrates. The relationship between ontogeny and phylogeny has long been an intriguing question in comparative and evolutionary embryology [1] . Biogenetic law of Ernst Haeckel assumed a parallelism between ontogeny and phylogeny, and asserted that embryogenesis is a recapitulation of ancient organisms because all animals start their existence from a one-celled stage and develop into morula, blastula and then gastrula stages [2] , [3] . Although it is now widely accepted that embryogenesis cannot simply be a repetition of evolution, none of the alternative formulations has reached a consensus, even with contemporary evolutionary developmental ('evo-devo') theories [2] . For example, we still do not know how to explain the common early embryonic stages, such as the morula, blastula and gastrula, in evolutionary terms. Is this because earlier stages of embryogenesis tend to be more evolutionarily conserved? One of the major controversies, which are limiting the formulation of an evolutionary model of embryogenesis, is whether the earliest or organogenesis phase of the embryonic period is more resistant to evolutionary change and, hence, more conserved among vertebrate embryos ( Fig. 1 ). 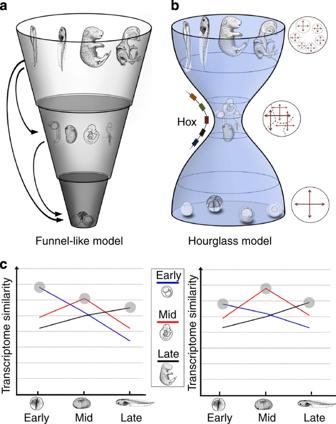Figure 1: The two major hypotheses about how developmental processes are conserved against evolutionary changes. In both models, embryogenesis proceeds from the bottom to the top, and the width represents the phylogenetic diversity of developmental processes, which are deduced from morphological similarities. (a) The funnel-like model predicts conservation at the earliest embryonic stage. During embryogenesis, diversity increases additively and progressively. This model is based upon the extreme case of developmental burden or generative entrenchment, in which the viability of any developmental feature depends on an earlier one (arrows). (b) The hourglass model predicts conservation of the organogenesis stage. Circles beside the model indicate inductive general features of signals observed during each stage. During this stage, a highly intricate signalling network is established consisting of inductive signals, including theHoxgenes11, which leads to conservation of the animal body plan12.Figure 1bwas adapted with permission from 11 and 12. (c) Hypothetical data supporting the funnel-like (left) and hourglass (right) models. For both examples, the transcriptome data ofM. musculusembryos (early, middle and late stages) were compared withX. laevisembryos (early, middle and late stages) in an all-to-all manner. The data, which are consistent with the funnel-like model, show that the transcriptome similarity is highest in the early versus early comparison (shaded point on the blue line; left). Data that are consistent with the hourglass model show that the transcriptome similarity is highest in the middle versus middle comparison (right). Figure 1: The two major hypotheses about how developmental processes are conserved against evolutionary changes. In both models, embryogenesis proceeds from the bottom to the top, and the width represents the phylogenetic diversity of developmental processes, which are deduced from morphological similarities. ( a ) The funnel-like model predicts conservation at the earliest embryonic stage. During embryogenesis, diversity increases additively and progressively. This model is based upon the extreme case of developmental burden or generative entrenchment, in which the viability of any developmental feature depends on an earlier one (arrows). ( b ) The hourglass model predicts conservation of the organogenesis stage. Circles beside the model indicate inductive general features of signals observed during each stage. During this stage, a highly intricate signalling network is established consisting of inductive signals, including the Hox genes11, which leads to conservation of the animal body plan12. Figure 1b was adapted with permission from 11 and 12. ( c ) Hypothetical data supporting the funnel-like (left) and hourglass (right) models. For both examples, the transcriptome data of M. musculus embryos (early, middle and late stages) were compared with X. laevis embryos (early, middle and late stages) in an all-to-all manner. The data, which are consistent with the funnel-like model, show that the transcriptome similarity is highest in the early versus early comparison (shaded point on the blue line; left). Data that are consistent with the hourglass model show that the transcriptome similarity is highest in the middle versus middle comparison (right). Full size image Haeckel's biogenetic law has been rehashed and can now be summarized as the concept that the highest conservation occurs at the earliest stage of embryogenesis [4] , [5] , [6] , [7] , which is the funnel-like model ( Fig. 1a ). Theoretical studies support this model by arguing that mutations or perturbations, which affect earlier stages in development, should be more likely to have widespread downstream effects, such as embryonic lethality, which are more difficult to be inherited [4] , [5] , [6] , [7] . In addition, molecular studies have suggested the existence of strong genomic constraints at the early stages of embryogenesis by showing the sequence conservation of genes, which are expressed during such phases [8] , [9] . Karl von Baer proposed a different idea that the highest morphological similarities can be found during mid-embryonic or organogenesis stages, such as the pharyngula stage [10] . Re-examination of this idea in terms of the morphological divergence in early embryogenesis, such as variations in cleavage, germ layer formation or gastrulation, has led to the development of the 'egg-timer' [11] and 'hourglass' models [11] , [12] ( Fig. 1b ). Two hypotheses have been proposed to provide a rationale for the conservation of mid-embryonic stages. One is that the spatial and temporal colinearity of the Hox gene cluster constrains the mid-embryonic stage; therefore, morphological diversification at this stage is unlikely [11] . Another hypothesis focuses on the peculiar modularity of developmental programs during mid-embryogenesis. Specifically, it proposes that intricate networks of both global and local inductive signals [12] during these stages make the development of different organ primordia highly interdependent. As a result, any change in the developmental events during these stages would increase the risk of mortality, and therefore, lead to evolutionary conservation by eliminating such changes. An important prediction of the hourglass model is the establishment of a 'phylotypic progression' or 'phylotype' in the mid-embryonic stages [11] , [12] , [13] , [14] , [15] . The phylotypic progression (or period) imposes constraints on morphological diversification; thereafter, it becomes the source of the basic body plan for each individual major taxon (or phylum). Some researchers have expanded the phylotype to include protostomes, calling it the 'zootype' [16] because similar expression patterns of Hox genes can be found among these organisms. Distinguishing between these two models of conservation during embryogenesis is important to explain how the basic body plan of vertebrates develops in an evo-devo context. The vertebrate body plan, which includes an overt head, trunk with segmented vertebrae and a segmented pharynx, is defined as a set of shared morphological traits of adult vertebrates and is assumed to originate from a conserved pattern of embryogenesis. However, if the 'funnel-like' model were held true, then this assumption would need to be reconsidered. In this case, it should be possible to distill the morphological elements of the vertebrate body plan into even simpler morphological elements, such as those seen in early embryos, because this model predicts that the greatest morphological similarity occurs at the earliest developmental stage. Owing to the difficulty in evaluating evolutionary distances between embryos of different species quantitatively, the identification of the most conserved embryonic stage remains controversial [8] , [9] , [17] , [18] , [19] , [20] , [21] . For example, there does not seem to be any consensus about how the difference between qualitatively different morphological traits, such as somites, pharyngeal arches and cleavage patterns, should be quantified [17] , [20] . Although some studies on the sequences of expressed genes [8] , [9] , [18] have made progress in quantitative comparisons, no study has succeeded in analysing the conservation of gene expression profiles between different vertebrates. As animal development can be interpreted as a process of producing various cell types from a single fertilized egg, comparing the cell type composition in vertebrate embryos could help clarify the most conserved stages. Thus, an analysis of the expression levels of various 'marker genes' in whole embryos may be a valuable approach. However, as this approach includes some research bias in selecting appropriate marker genes, we decided to use global comparisons of gene expression profiles. Briefly, we aimed to identify the conserved stages of embryogenesis and test the 'funnel-like' and 'hourglass' models by comparing the transcriptomes of whole embryos as a reflection of the composition of orthologous cell types ( Fig. 1c ). Here, we show for the first time that the highest conservation in gene expression profiles of vertebrate embryos occurs in the pharyngular embryo (embryos with pharyngeal arch), which is considered to be the source of the basic body plan of vertebrates in comparative morphology. Furthermore, our data not only support the hourglass model but also intensifies the debate on the decreasing divergence detected during early to mid-embryonic stages. 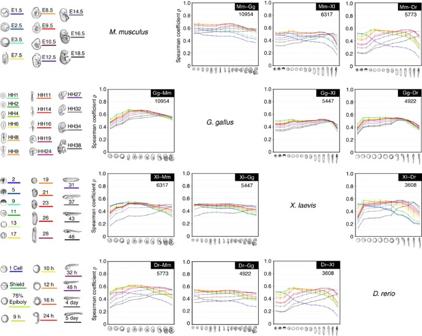Figure 2: Transcriptome similarities of different embryos. Spearman correlation coefficients (ρ) of the transcriptome data from pairs of embryos from different species at different developmental stages. Higher ρ values indicate higher transcriptome similarity. The sampled stages are shown on the left. Different coloured lines indicate different developmental stages. For example, in the chart for the Dr–Xl comparison, the left end of the blue line indicates the Spearman correlation coefficients of a one-cellD. rerioembryo and a stage twoX. laevisembryo. As the comparison proceeds to later developmental stages ofX. laevis, or to the right of the blue line, the Spearman correlation coefficients decrease. Note that the ρ scores calculated for the early versus early stages (left part of the blue lines in each graph) are not the highest. The number in the upper right corner of each chart indicates the number of orthologous genes, which were used to calculate the transcriptome similarities. Error bars indicate s.d. Mid-embryonic stages show higher transcriptome similarity than other stages The transcriptome similarities, which can be regarded as a possible estimate of evolutionary distance, of early to late embryos from four vertebrate species, namely mouse ( Mus musculus ), chicken ( Gallus gallus ), African clawed frog ( Xenopus laevis ) and zebrafish ( Danio rerio ), are shown in Figure 2 . As it is impossible and unrealistic to define developmentally equivalent stages between different animal species, we compared the transcriptomes of embryo stages in an all-to-all manner (for example, the left end of the blue line in the Dr–Xl panel of Fig. 2 shows that, the transcriptomes of the one-cell stage, D. rerio and the stage 2 of X. laevis pair have the highest similarity, whereas the right side of the blue line shows that the similarity decreases when compared with the later developmental stages of X. laevis ). These comparisons allowed us to deduce inter-species correspondences for various developmental stages ( Supplementary Fig. S1 ) and demonstrated that none of the single stages have higher similarity than any others. Figure 2: Transcriptome similarities of different embryos. Spearman correlation coefficients (ρ) of the transcriptome data from pairs of embryos from different species at different developmental stages. Higher ρ values indicate higher transcriptome similarity. The sampled stages are shown on the left. Different coloured lines indicate different developmental stages. For example, in the chart for the Dr–Xl comparison, the left end of the blue line indicates the Spearman correlation coefficients of a one-cell D. rerio embryo and a stage two X. laevis embryo. As the comparison proceeds to later developmental stages of X. laevis , or to the right of the blue line, the Spearman correlation coefficients decrease. Note that the ρ scores calculated for the early versus early stages (left part of the blue lines in each graph) are not the highest. The number in the upper right corner of each chart indicates the number of orthologous genes, which were used to calculate the transcriptome similarities. Error bars indicate s.d. Full size image Pharyngular embryos have the highest transcriptome similarity As shown by the pairwise species comparisons in Figure 2 , embryonic stages ranging from the neurula to the late pharyngula tended to have highly similar transcriptomes, although the stage of highest similarity differed among the pairs of species. On the other hand, the transcriptomes from the cleavage to blastula and later stages were less similar. Importantly, these results did not change with different methods of normalization or calculating transcriptome similarity (Methods and Supplementary Fig. S2 ). These results are consistent with the predictions of the hourglass model, but not with that of the funnel-like model. However, the conserved stages in these pairwise species comparisons simply reflect the most conserved embryonic stage within each clade (for example, the amniote-conserved stage in the mouse–chicken comparison) and may not reflect the commonly conserved stage in Vertebrata. As these models aim to explain the stage-dependent conservation of vertebrate embryos in general, we further analysed the overall or average similarities of transcriptomes of representative embryonic stages of the four species. Similar to the pairwise comparisons ( Fig. 2 ), the transcriptome similarities among the representative stages were the highest for the pharyngula ( Fig. 3a,b ). The results also did not show any significant change with different methods of normalization or calculating transcriptome similarity. 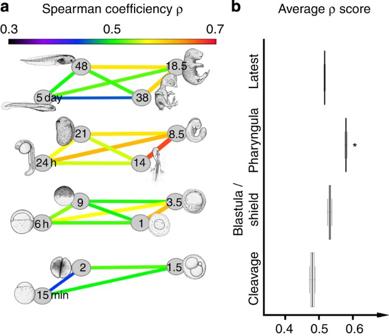Figure 3: Higher transcriptome similarities among representative pharyngula stages. (a) Spearman correlation coefficient (ρ) of the expression profiles of 1,573 core orthologues from representative stages of cleavage, blastula/shield, pharyngula (defined here as the stage of onset of pharyngeal arch formation) and late-stage embryos. Numbers or text in the grey spheres indicate the stage of each species. The colours of the lines, which connect each stage, reflect the ρ value, according to the colour gradient shown at the top. (b) Box (quantile) plot of the ρ scores of representative stages, which were evaluated with hierarchical Bayes-based, Kruskal–Wallis analysis of variance tests (P=1.9×10−12). The asterisk indicates that the ρ scores of the pharyngula stages were significantly higher than that of the cleavage, blastula/shield or late embryo stages (Wilcoxon test corrected α=0.0017). Figure 3: Higher transcriptome similarities among representative pharyngula stages. ( a ) Spearman correlation coefficient (ρ) of the expression profiles of 1,573 core orthologues from representative stages of cleavage, blastula/shield, pharyngula (defined here as the stage of onset of pharyngeal arch formation) and late-stage embryos. Numbers or text in the grey spheres indicate the stage of each species. The colours of the lines, which connect each stage, reflect the ρ value, according to the colour gradient shown at the top. ( b ) Box (quantile) plot of the ρ scores of representative stages, which were evaluated with hierarchical Bayes-based, Kruskal–Wallis analysis of variance tests ( P =1.9×10 −12 ). The asterisk indicates that the ρ scores of the pharyngula stages were significantly higher than that of the cleavage, blastula/shield or late embryo stages (Wilcoxon test corrected α=0.0017). Full size image As these representative stages were chosen arbitrarily, we performed a more rigorous and robust analysis using total sum distance analysis to identify the most conserved stages among four species. Although the combinations of embryos with the highest transcriptome similarity varied according to the methods that were used for normalization and calculating transcriptome similarity, all of these data contained the following combinations of embryonic stages ( Supplementary Table S1 ): M. musculus embryonic gestation day (E) 9.5+ G. gallus Hamburger-Hamilton (HH) stage 16+ X. laevis stage 28+ D. rerio 24 h postfertilization (hpf) and M. musculus E9.5+ G. gallus HH16+ X. laevis stage 31+ D. rerio 24 hpf. Interestingly, these stages showed most of the characteristics of Ballard's definition of the pharyngula stage, which is generally regarded as the phylotypic stage of vertebrates [23] : a head, pharyngeal arches, somites, neural tube, epidermis but no hair or feathers, kidney tubules and longitudinal kidney ducts but no metanephros, a heart with chambers, at least a transient cloaca, no middle ear, no gills on the pharyngeal segments, no tongue and no penis or uterus ( Supplementary Table S2 ). In addition, these stages overlapped with the timing of Hox gene expressions along the antero-posterior axis [16] , which is considered to be one of the molecular characteristics of the vertebrate phylotype [11] , [16] , [24] . Genes with conserved expression during the phylotypic period To further investigate the molecular characteristics of the most conserved developmental stages, we identified genes that showed conserved expression during the above stages, but excluded those that were expressed constitutively throughout embryogenesis. This resulted in the identification of 109 orthologous (see Supplementary Data 1 ) and 182 coorthologous gene sets (see Supplementary Data 2 ). In addition to the Hox genes, we also found many genes that are involved in cell–cell signalling and interactions (for example, Fzd2, ptch2, Sema3d, FGFRL1 and Dscaml), transcription factors (for example, FoxG1, Pax6, myf6, Tbox20, Islet1, Emx2 and Klf2), and secreted morphogens or growth factors (for example, Dkk, FGF8, Angpt1 and INS; see Supplementary Data 1 ). Notably, within the 109 orthologous gene sets, genes with similar expression profiles contained higher proportions of development-related genes (defined by gene ontology) than that with different expression profiles ( Supplementary Fig. S3 ). Unlike several recent studies that support the funnel-like model [8] , [9] , our results showed that the mid-embryonic stages are the most conserved vertebrate developmental stages in terms of comparative transcriptomes ( Figs 2 and 3 ), which is consistent with the hourglass model and the phylotype hypothesis. Currently, even among those that support the hourglass model, there is no consensus on which developmental stage or features characterize the morphological aspect of the phylotypic period (pharyngula [23] , early somite [15] or tailbud stage [16] ). Our mathematical analyses allowed us to identify combinations of conserved stages, in terms of transcriptomes, within four different vertebrate species, such as M. musculus E9.5+ G. gallus HH16+ X. laevis stage 28 and 31+ D. rerio 24 hpf. Although X. laevis stage 28 corresponds to the tailbud stage, all of the other stages seem to be best described as the pharyngula stage. Although this stage is an attractive candidate for the phylotypic period of vertebrates, it does not mean that all vertebrate embryos pass through a morphologically identical embryonic stage [25] . Instead, it appears to be a stage that involves minimal heterochronic changes or a stage that shows the highest common factor of developmental processes [20] , [26] . Previous studies, which have used gene expression approaches [8] , [9] , [18] , [27] , have mainly focused on the primary sequences of expressed genes. In contrast, our focus in this study was the similarity of regulated gene expression, and this is in concordance with the well-known evo-devo hypothesis that modifications of gene regulatory networks have fundamental roles in morphological evolution [28] . The discrepancies in previous sequence-based studies were probably because of the scarcity of gene expression data for vertebrate embryos; therefore, most of those studies only analysed a single species. In fact, we did not find any statistically significant relationship between embryonic stages and the 'protein distance' of expressed genes. Moreover, even though some of the data were weakly correlated with low statistical significance (0.1< P <0.05), none of these correlations was consistent among the four species ( Supplementary Fig. S4 ). Slack et al . [16] provided an important insight into the embryogenesis of the common bilaterian ancestor by proposing that the 'zootype' is most clearly expressed during the phylotype. Therefore, we analysed whether the phylotypic period is the most conserved embryonic stage across all the bilaterians (albeit derived to some extent) at the transcriptome level. Our preliminary analysis with Anopheles gambiae did not contradict this viewpoint; we found that high transcriptome similarities between A. gambiae and vertebrate embryos occurred at the mid-embryonic stages (segmentation stage for A. gambiae and neurula to pharyngular stages for vertebrates, see Supplementary Fig. S5 ). The segmentation stage is an attractive candidate for the zootype period; however, our analysis of the total sum distance did not provide conclusive evidence for this conclusion. A similar analysis with more protostomes is needed to confirm this conclusion and develop a unified understanding of the last common bilaterian ancestor or Urbilaterian [29] . There might be some disagreement about the relevancy of our molecular-based approach to test the two morphologically established models (the funnel-like and hourglass model). However, the central argument of the two models is to elucidate the conserved developmental programs of vertebrates. Morphological similarity has been a limited resource for estimating the evolutionary distance between various developmental programs, but inherited entity is not morphological information. Therefore, our approach might be better suited for verifying the two models. Another possible disagreement could be that the conservation of mid-embryonic stages is a 'by-product' of a modified version of the funnel-like model. In other words, embryonic divergence and the addition of early divergence by maternal effect genes might point misleadingly to mid-embryonic conservation. However, regardless of the mRNA source, the detection of divergence in the earliest developmental stages is unavoidable. In addition, the conserved stages that we identified in our analysis seem to occur too late to be explained by this idea [30] (for example, in mice, maternal RNAs and proteins are degraded by E3.5 (ref. 31 )). One shortcoming of our study is that we could not include basal vertebrate lineages, such as cyclostomes. Thus, there is still a possibility that the conserved stages, which we identified in our analysis, are gnathostome-specific at best. One unanswered question in this field is how pharyngular stages became conserved. Even with our data, this may be a difficult question to answer because the conservation of mid-embryonic stages observed here would be the product of evolution on a geological timescale and might have involved various effects, including natural selection, biased mutations, limited flexibility of embryogenesis and genetic drift. Nevertheless, several possible explanations have been proposed, such as an intricate network of developmental signals [12] , developmental burden [5] or natural selection that acts on final structures of primordial found specifically at these stages [5] . However, as many 'developmental toolkit' genes [22] , including Hox genes, are expressed in all putative phylotypic period embryos, it is possible that these genes are part of a developmental network, which is resistant to change, and could be a source of developmental constraint. Regardless of the mechanism of the conservation of mid-embryonic stages, a certain characteristic of embryogenesis seems to be required to explain the waist of the hourglass model. In other words, how did vertebrate embryos allow the early developmental stages to diverge while keeping the following stage essentially unchanged? For example, in spite of considerable phylogenetic divergence in the mechanisms of vertebrate germ layer formation and gastrulation [32] among the four species we analysed, all these embryos pass through the conserved pharyngula stage. How did vertebrates establish divergence of early embryogenesis while keeping pharyngular stages conserved? One reasonable deduction from this observation is that early vertebrate embryogenesis reduces the developmental fluctuations, which tend to occur around these stages, much like earthquake-resistant buildings that are built with the 'flexible structure' [33] . This stabilizing role of early-to-mid developmental process is consistent with a prediction of the theory called 'isologous diversification for cell differentiation' in complex systems biology [34] . In addition, it is important to note that developmental stages might be more or less uncoupled from each other, which would allow evolutionary changes to be introduced rather independently; indeed, adults and larvae are said to evolve and diverge independently [35] . Our approach in this study is a novel method for quantitatively estimating the similarity between embryonic stages or putative evolutionary distances in terms of the transcriptome, which allows the conserved stages of vertebrates to be identified. In addition, it reveals the approximate correspondences among developmental timetables, which are usually out of sync in actual time ( Supplementary Fig. S1 ). Further refinement of this methodology with other molecular techniques, such as RNA sequencing at tissue-level resolution, may allow us to address heterochrony at a molecular level. Collection of staged embryos and RNA samples Whole embryos (except for extraembryonic membranes) of M. musculus ( Mm ; C57BL/6), G. gallus ( Gg ), X. laevis ( Xl ) and D. rerio ( Dr ) were staged and collected according to the normal criteria [36] , [37] , [38] , [39] . At least three embryos of the same stages were pooled and homogenized, and total RNA was extracted to make staged samples for microarray analyses. To represent the general population of each developmental stage, non-littermate embryos were collected and used for biological replications (two or more replications for each stage). All the animal experiments were carried out in accordance with the guidelines of our Institutional Animal Ethics Committee. Criteria for orthologous genes Basic Local Alignment Search Tool (BLAST) searching (E-value <1e–5) was applied to the non-redundant proteome of each organism downloaded from the National Center for Biotechnology Information (NCBI) website ( ftp://ftp.ncbi.nih.gov/genomes/ ) and the EMBL Ensembl website ( http://www.ensembl.org/ ). Pairs of genes with reciprocal best BLAST hit (RBBH) were defined to be orthologues. Core orthologues were defined by the 1-1-1-1 version of RBBH within the proteomes of Mm, Gg, Xl and Dr. For identifying orthologous gene groups, we took advantage of the orthoMCL program [40] , because the RBBH-based core orthologues exclude paralogous genes. In brief, orthoMCL improves on RBBH by including the detection of orthologues and paralogues, a normalization step and Markov clustering. Microarray data For each sample, total RNA was labelled and hybridized to a species-specific Affymetrix GeneChip (Mouse Genome 430 2.0 Array, Chicken Genome Array, X. laevis Genome 2.0), according to the manufacturer's instructions (Affymetrix). The raw CEL data for each species were normalized by either MAS5, PMdChip or gcRMA software within species, to confirm that our conclusions were not affected by the method of normalization. MAS5 normalized data were used for the figures. For inter-species comparisons of orthologous gene expressions, RBBH was applied to each organism's non-redundant proteome downloaded from the NCBI website ( ftp://ftp.ncbi.nih.gov/genomes/ ) and the EMBL Ensembl website ( http://www.ensembl.org/ ). We further evaluated their expression values from corresponding GeneChip probe sets defined by Affymetrix annotation files. Numbers of orthologous gene expressions that were comparable one-to-one to species were as follows: 5,447 genes for Gg_versus_Xl, 4,922 genes for Gg_versus_Dr, 10,954 genes for Mm_versus_Gg, 5,773 genes for Mm_versus_Dr, 6,317 genes for Mm_versus_Xl and 3,608 genes for Dr_versus_Xl; while 1573 1-1-1-1 RBBH orthologues were comparable within these GeneChips. These expression data were submitted to the EMBL-EBI ArrayExpress database ( http://www.ebi.ac.uk/microarray-as/ae/ ) under accession numbers E-MTAB-366 , E-MTAB-368 and E-MTAB-369 . Mouse microarray data of E1.5–3.5 wild-type embryos and zebra fish microarray data of wild-type embryos were downloaded from ArrayExpress (E-GEOD-11687 [41] for the mouse and E-TABM-33 for the zebra fish). Evaluation of transcriptome similarity The Pearson correlation coefficient ( r ), Spearman correlation coefficient (ρ), total Euclidean distance ( D E ) and total Manhattan distance ( D M ) were used independently to evaluate transcriptome similarity between different samples. In brief, higher values of r and ρ, and lower values of D E and D M indicate higher transcriptome similarity. For calculating these values, log 2 transformed expression scores were used (the Spearman correlation coefficient further transforms the expression value into rank-transformed values). Euclidean and Manhattan distances were calculated after performing a Quantile normalization to meet the assumptions of these methods. Total sum distance analysis was performed as follows: we first made data sets consisting of 29,700 combinations of stages by selecting one developmental stage per species (number of combinations=11 Mm_stages×15 Gg_stages×15 Xl_stages×12 Dr_stages=29,700), then calculated 6 transcriptome similarities among the 4 embryos ( 4 C 2 =6) and summed these similarities. These total sum distance scores were tested by non-parametric statistical test. Statistical tests An alpha level of 0.01 was accepted for statistical significance throughout the analyses, and a Bonferroni correction was applied when performing multiple comparisons to avoid an inflated type I error rate. Values of correlation coefficients (Spearman or Pearson) were regarded as valid only when the comparison was confirmed to have a significant correlation by a test of non-correlation. The Welch two-sample t -test was used for two-sample comparison when the data passed the Kolmogorov–Smirnov test for normal distribution. Software and computation environment Data processing and command pipelining were done using customized Perl scripts, Perl modules and C shell scripts. BLAST searches were carried out using the stand-alone NCBI-BLAST [42] . Statistical analyses and plottings were performed using R ( http:/www.R-project.org/ ) [43] , including the R package Bioconductor [44] for microarray normalization and preprocessing. Cytoscape ( http://www.cytoscape.org/ ) [45] was used for network visualization. Heavy calculations were performed using the RIKEN Integrated Cluster of Clusters supercomputer of the RIKEN Advanced Centre for Computing and Communication, Saitama, Japan. Accession codes: Expression data were submitted to the EMBL-EBI ArrayExpress database ( http://www.ebi.ac.uk/microarray-as/ae/ ) under accession numbers E-MTAB-366 , E-MTAB-368 and E-MTAB-369 . How to cite this article: Irie, N & Kuratani, S. Comparative transcriptome analysis reveals vertebrate phylotypic period during organogenesis. Nat. Commun. 2:248 doi: 10.1038/ncomms1248 (2011).